Field-effect reconfigurable nanofluidic ionic diodes Several types of nanofluidic devices based on nanopores and nanochannels have been reported to yield ionic current rectification, with the aim to control the delivery of chemical species in integrated systems. However, the rectifying properties obtained by existing approaches cannot be altered once the devices are made. It would be desirable to have the ability to modulate the predefined properties in situ without introducing external chemical stimuli. Here we report a field-effect reconfigurable nanofluidic diode, with a single asymmetrically placed gate or dual split-gate on top of the nanochannel. The forward/reverse directions of the diode as well as the degrees of rectification can be regulated by the application of gate voltages. Compared with the stimuli-responsive tuning of the rectification properties, the electrostatic modulation offers a fully independent and digitally programmable approach for controlling the preferential conduction of ions and molecules in fluids. This device would serve as a building block for large-scale integration of reconfigurable ionic circuits. With applications ranging from biosensing to the control of molecular transport, synthetic nanopores and nanochannels are the focus of growing scientific interest [1] . Analogous to a solid-state semiconductor diode for regulating the flow of electrons/holes to one preferential direction, nanofluidic diodes are being developed to achieve the rectified ionic transport-ions favourably move in one direction and are inhibited in the opposite direction. Such rectification effect is of great importance owing to its relevance to biological ion channels [2] . Moreover, ionic diodes, together with ionic transistors [3] , [4] , [5] , [6] , [7] , [8] , [9] represent the key building blocks for ionic circuits [10] , [11] , which would allow for regulating [6] , sensing [12] , concentrating [13] and separating [14] ions and molecules in electrolyte solutions, mimicking voltage-gated ion channels in a variety of biological systems. Several nanofluidic platforms based on nanopores and nanochannels were reported to produce ionic current rectification by symmetry breaking [15] in geometries [16] , [17] , [18] , [19] , surface charge distributions (either intrinsic material properties [20] , [21] or chemically modified properties [22] , [23] ), bath concentrations [24] , or a combination of them, for example, by positively and negatively patterning charged regions in conical nanopores [25] . Nevertheless, it has not been possible to change the predefined rectifying properties obtained by these approaches once the devices are made. Although several externally tunable methods have been proposed so far, most of them aim to alter the nanochannel wall property by introducing external chemical stimuli, for example, hydronium ions (pH) [26] , [27] , [28] , enzymes [29] and polyvalent cations [30] . All these methods require changing the native environment of the solution being transported. Contrary to the chemical stimuli-responsive schemes, an electric field normal to the nanochannel walls is able to enhance or diminish the ionic concentrations near the surface in situ [3] , [4] , [5] , [6] , [7] , [8] , [9] , resembling the carrier number modulation in a metal-oxide-semiconductor field-effect transistor. Here we report a field-effect reconfigurable ionic diode by asymmetrically modulating the cation/anion ratios along the nanochannel. The field-effect approach requires no solution replacement and allows large-scale integration for more complex functions. A key feature of our device is that it allows the post-fabrication reconfiguration of the diode functions, such as the forward/reverse directions as well as the rectification degrees. These results may lead to the creation of reconfigurable ionic circuits, an ionic counterpart of the electronic field-programmable gate array. 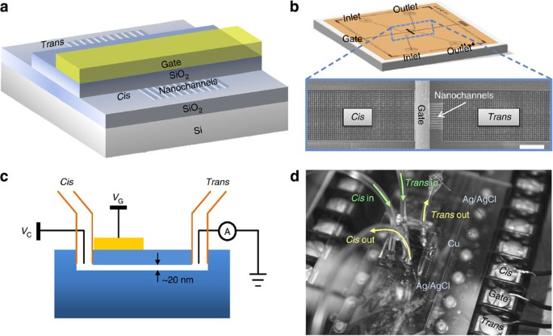Figure 1: Device structure and experimental setup. (a) Schematic of the nanofluidic FERD. (b) Sketch of the planar layout for the assembled device. Two microfluidic channels deliver the electrolyte solutions to theCisandTransreservoirs, formed by SiO2trenches with supporting pillars, as shown in the magnified scanning electron microscope (SEM) image. The scale bar in the SEM image is 100 μm. There are 11 parallel nanochannels connectingCisandTransreservoirs. The supporting pillars prevent the microfluidic polydimethylsiloxane from collapsing into the reservoirs. (c) Schematic of the electrical and fluidic connection configurations. The electrical contacts are made of Ag/AgCl electrodes and are integrated with the connecting tubes, serving as a low resistive loss contact.VGandVCdenotes the voltage on the gate andCis, respectively. TheTransside is referenced as ground in all measurements in this study. The whole setup is placed in a Faraday cage to shield the electrostatic noise. (d) Photograph of a FERD device with electrical and fluidic connections. Device structure The schematic structure of the nanofluidic field-effect reconfigurable diodes (FERD), and the experimental setup is illustrated in Figure 1 . The FERD is a three-terminal device that has a similar structure to a nanofluidic field-effect transistor (FET) [6] , [7] , yet with a critical difference that the gate electrode of FERD is asymmetrically located near one of the microfluidic reservoirs. The control devices with gate electrodes sitting symmetrically along the nanochannel were also fabricated on the same silicon wafer. We used a sacrificial layer method to produce the nanochannels (20 nm in height) with a novel 'bond-followed-by-etch' scheme, which completely avoids the nanochannel collapse problem encountered in conventional 'etch-and-bond' schemes ( Supplementary Fig. S1 and Supplementary Methods ). To make a consistent notion in the following discussion, we denote the microfluidic reservoir that is close to the gate electrode as Cis (C) and the other reservoir far away from the gate electrode as Trans (T). Figure 1: Device structure and experimental setup. ( a ) Schematic of the nanofluidic FERD. ( b ) Sketch of the planar layout for the assembled device. Two microfluidic channels deliver the electrolyte solutions to the Cis and Trans reservoirs, formed by SiO 2 trenches with supporting pillars, as shown in the magnified scanning electron microscope (SEM) image. The scale bar in the SEM image is 100 μm. There are 11 parallel nanochannels connecting Cis and Trans reservoirs. The supporting pillars prevent the microfluidic polydimethylsiloxane from collapsing into the reservoirs. ( c ) Schematic of the electrical and fluidic connection configurations. The electrical contacts are made of Ag/AgCl electrodes and are integrated with the connecting tubes, serving as a low resistive loss contact. V G and V C denotes the voltage on the gate and Cis , respectively. The Trans side is referenced as ground in all measurements in this study. The whole setup is placed in a Faraday cage to shield the electrostatic noise. ( d ) Photograph of a FERD device with electrical and fluidic connections. Full size image Nanochannel characterization We first carried out experiments on the electrical characterization ( Supplementary Fig. S2 ) of the nanochannels with the gate terminal floating. By measuring the nanochannel conductance as a function of KCl concentration ( C b ), we observed a linear dependence of channel conductance on C b in the high-concentration regime and a conductance plateau in the low-concentration regime ( Fig. 2 ). The transition concentration is around 1 mM, at which the corresponding Debye screening length (λ D ) is around 10 nm, equal to half of the designed nanochannel height. This behaviour confirms a surface-charge governed ionic transport property [31] , [32] . By knowing the dimensions of the lithographically defined channels, the surface charge density (σ s ) can be derived by fitting the experimental data ( Supplementary Methods ). We tested two individual devices fabricated on the same wafer but with different channel width W (2 μm×11 and 3 μm×11, respectively). Both of them can be well fitted by a same σ s (−2 mC m −2 ), suggesting the surface properties remain consistent and reliable after the 'bond-followed-by-etch' process. This σ s value is close to those reported with the plasma-enhanced chemical vapour deposition SiO 2 (~−4.5 mC m −2 ) [20] , [24] . 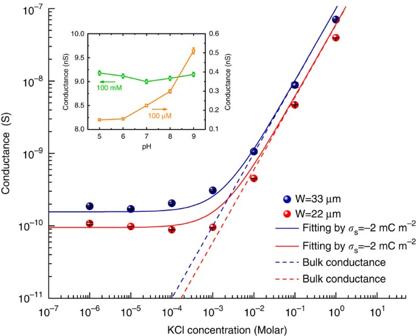Figure 2: Measured conductance as a function of KCl concentrations for two devices. Both devices were fabricated using the identical process on a same wafer with gate terminal floating (Blue:W=33 μm,L=100 μm,H=20 nm. Red:W=22 μm,L=100 μm,H=20 nm). Solid lines are the fitting curves with σs=−2 mC m−2. Dashed lines are the bulk prediction that deviates from the experimental data in the low ionic concentration region. The error bars correspond to ten measurements and are smaller than the size of the symbol used. Inset shows the pH dependence of channel conductance at two electrolyte concentrations ([KCl]=100 μM and [KCl]=100 mM). The pH of the electrolyte solution is adjusted by adding hydrochloric acid or potassium hydroxide into 100-μM phosphate buffers. The error bars correspond to ten measurements. Figure 2: Measured conductance as a function of KCl concentrations for two devices. Both devices were fabricated using the identical process on a same wafer with gate terminal floating (Blue: W =33 μm, L =100 μm, H =20 nm. Red: W =22 μm, L =100 μm, H =20 nm). Solid lines are the fitting curves with σ s =−2 mC m −2 . Dashed lines are the bulk prediction that deviates from the experimental data in the low ionic concentration region. The error bars correspond to ten measurements and are smaller than the size of the symbol used. Inset shows the pH dependence of channel conductance at two electrolyte concentrations ([KCl]=100 μM and [KCl]=100 mM). The pH of the electrolyte solution is adjusted by adding hydrochloric acid or potassium hydroxide into 100-μM phosphate buffers. The error bars correspond to ten measurements. Full size image AS the surface charge can be modified by changing the solution pH, we further tested the pH dependence of the nanochannel conductance at fixed KCl concentrations (inset of Fig. 2 ). At high KCl concentrations (100 mM), changing the pH value has negligible impact on the channel conductance, whereas at low KCl concentrations (100 μM), pH has a pronounced impact. This behaviour can be well explained by surface charge governed transport property. At high ionic concentrations, the double layer conductance (which is regulated by pH values) is overwhelmed by the bulk conductance. Therefore, the channel conductance will not change by varying pH. At low KCl concentrations, the channel conductance is dominated by the double layer and is thus pH-dependent. As [H + ] for a given electrolyte concentration decreases, the number of SiO surface charges increases [33] . 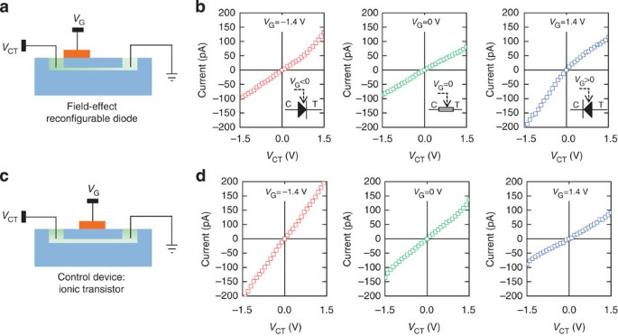Figure 3: Current-voltage (I-V) curves for the FERD devices with different gate voltage (VG) polarities. (a) Testing configurations for the FERD device. (b) I-V curves for FERD devices (W=2 μm×11,L=100 μm,H=20 nm) using a 100-μM KCl solution. An apparent gate voltage-controlled rectifying property is observed. The inset symbols schematically show the forward direction switched on positive and negative gate voltages. (c) Testing configurations for the control transistor device. (d)I-Vcurves for the control device (W=3 μm×11,L=100 μm,H=20 nm) using a 100-μM KCl solution. Gate voltage can modulate the channel conductance but no rectifying property is observed. Field-effect reconfigurability After verifying that the device conductance is indeed governed by the ion transport in the nanochannels (instead of leakage paths), we went on to investigate the field-effect tunability of the three-terminal FERD devices using electrical configurations shown in Figure 3a . The channel current as a function of Cis to Trans voltage ( V CT ) was measured under various gate voltages ( V G ). Figure 3b shows the representative current-voltage ( I – V ) curves obtained with V G of different polarities, using a 100-μM KCl solution. A clear gate-voltage controlled rectifying property is observed. At V G =0 (middle panel, Fig. 3b ), the I - V curve is symmetric with respect to the origin. At a negative gate voltage (left panel, Fig. 3b ), the ionic current in the positive V CT regime is higher than that in the negative V CT regime. While at a positive gate voltage (right panel, Fig. 3b ), the negative V CT conducts more ionic current than the positive V CT . Consequently, it is possible to switch the preferential direction of the ionic flow via adjusting the external gate voltage, a novel mechanism of nanofluidic control that has never been shown before. Figure 3: Current-voltage (I-V) curves for the FERD devices with different gate voltage ( V G ) polarities. ( a ) Testing configurations for the FERD device. ( b ) I-V curves for FERD devices ( W =2 μm×11, L =100 μm, H =20 nm) using a 100-μM KCl solution. An apparent gate voltage-controlled rectifying property is observed. The inset symbols schematically show the forward direction switched on positive and negative gate voltages. ( c ) Testing configurations for the control transistor device. ( d ) I - V curves for the control device ( W =3 μm×11, L =100 μm, H =20 nm) using a 100-μM KCl solution. Gate voltage can modulate the channel conductance but no rectifying property is observed. Full size image We note that an electric potential barrier will develop at the micro/nano channel interface [34] , which is analogous to a potential barrier at a heterojunction in semiconductor devices due to a work function difference [35] . This interfacial barrier is indeed a negligible effect in our FERD devices and is not responsible for the voltage tunable rectifying property ( Supplementary Fig. S3 ). This conclusion is further verified by the I–V characteristics of the control devices (with symmetrically placed gate electrodes), schematically shown in Figure 3c . The major structural difference between the FERD devices and the control devices is the location of the gate terminal. No rectifying features are observed for the control device, which exhibits a symmetric I - V relationship for all V G polarities ( Fig. 3d ). The control device actually shows a typical p -channel transistor behaviour, where the conductance of the nanochannel is modulated by the field effect. In a negatively charged SiO 2 nanochannel, cations are the majority carriers, which are expected to increase or decrease when subjected to negative or positive electrostatic potentials, respectively. Therefore, the channel conductance will be enhanced at a negative V G and suppressed at a positive V G . From the comparison of the FERD and the control devices, we conclude that it is indeed the asymmetric positioning of the gate electrode that introduces the rectifying behaviour, whose favourable direction is not fixed but switchable via a gate potential. Qualitative analysis To understand the asymmetrical-gate controlled nanofluidic diodes, we developed a qualitative interpretation by looking at the change of the transient drift current of both cations and anions inside the nanochannel immediately after V CT bias is applied with different V G polarities ( Fig. 4a ). Because the ionic concentration distributions cannot change instantly, they remain the same as the steady state during this transient period. As a result, the diffusion current is not considered. 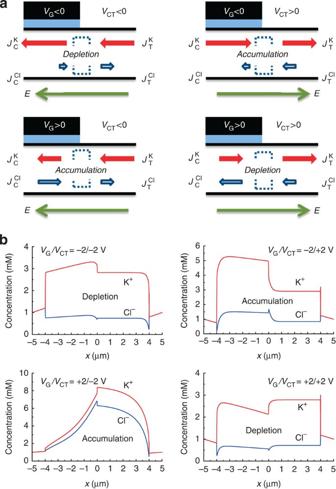Figure 4: Qualitative and quantitative analysis of the nanofluidic FERD. (a) Schematic diagram of cation and anion fluxes under various conditions. The solid red and the empty blue bars represent cation and anion concentrations as well as the corresponding current flux. The length of the bars depicts their amount (not to scale). The resulting ion depletion or accumulation taking place in the centre junction of the nanochannel at steady state can be obtained by comparing the amount of ion fluxes flowing into and away from the dashed box. (b) Quantitatively calculated steady state profiles of the ion concentrations along the channel length under differentVCTandVGpolarities at 1 mM KCl. The averaged K and Cl concentrations is calculated by, whereHis the channel height. The surface charge density used in the calculation isσs=−2 mC m−2. The solid and empty bars inside the nanochannels in Figure 4a correspond to the cation and anion concentrations, respectively. The length of the bars depicts the amount of the ionic concentration as well as the drift current (because the drift current is linearly proportional to the ionic concentrations). According to the Kirchhoff's current law, the sum of currents flowing into any node should be equal to the sum of currents flowing out of that node, we get . Therefore, the length sum of the two bars in each side of the channel should be equal. Figure 4: Qualitative and quantitative analysis of the nanofluidic FERD. ( a ) Schematic diagram of cation and anion fluxes under various conditions. The solid red and the empty blue bars represent cation and anion concentrations as well as the corresponding current flux. The length of the bars depicts their amount (not to scale). The resulting ion depletion or accumulation taking place in the centre junction of the nanochannel at steady state can be obtained by comparing the amount of ion fluxes flowing into and away from the dashed box. ( b ) Quantitatively calculated steady state profiles of the ion concentrations along the channel length under different V CT and V G polarities at 1 mM KCl. The averaged K and Cl concentrations is calculated by , where H is the channel height. The surface charge density used in the calculation is σ s =−2 mC m −2 . Full size image When the gate potential is negative (upper row in Fig. 4a ), the cation concentration immediately beneath the gate electrode is enhanced by the electrostatic attraction. With a negative V CT (upper left panel, Fig. 4a ), anions are driven towards the Trans side and the cations towards the Cis side, as indicated by the arrows. Under such a circumstance, the amount of the cation/anion flux flowing out of the centre junction of the nanochannel is larger than that flowing into it. As a result, when the system reaches the steady state again, the ions in the channel centre will be depleted, resulting in a depletion region with a lower conductance. Conversely, with a positive V CT bias (upper right panel, Fig. 4a ), the flow directions of the ions are reversed. More ions flow into the centre junction of the nanochannel while fewer ions flow out. This causes an accumulation of ions in the nanochannel and hence an increase of steady state conductance. Therefore, rectification of ionic transport is established and the preferential ionic current flow direction is from the Cis side to the Trans side when V G <0. When a positive gate voltage is imposed (lower row in Fig. 4a ), the cation concentration near the Cis side of the nanochannel is reduced by the electrostatic repulsion. Following the same analysis, it is obvious to conclude that a negative V CT conducts more ionic current than a positive V CT of the same magnitude. As a result, rectification of ionic current is also established, but the preferential ionic current direction is reversed as compared with the case of a negative gate potential. Quantitative analysis The quantitative analysis of the ion transport through the nanopores and nanochannels is generally calculated by concurrently solving the coupled Poisson–Nernst–Planck, and Navier–Stokes equations [36] , [37] , [38] , [39] , [40] . Since the contribution of electro-osmosis is usually very small compared with the diffusive components, the Navier–Stokes equations can be neglected [40] , [41] . We calculated the steady-state distributions of cation/anion concentrations by self-consistently solving the coupled Poisson–Nernst–Planck equations. To take into account the field effect arising from the externally imposed gate potential, the electric potential inside the gate dielectric is also solved simultaneously ( Supplementary Fig. S4 and Supplementary Methods ). The calculated concentration profiles under different V G and V CT polarities are shown in Figure 4b . The quantitative steady state ion profile agrees well with the qualitative transient analysis in Figure 4a . The ion enrichment and depletion effect at the micro/nano channel interface [13] is also observed in the calculated results ( x =±4 μm). This entrance effect contributes only a small portion of the total conductance and is not responsible for the field-effect-tunable rectifying property, as shown in Supplementary Figure S3 . Concentration dependence of the rectifying behaviour Interestingly, the field-effect reconfigurable rectifying behaviour shows a strong dependence on ionic concentrations. We recorded the I CT as a function of V CT for V G ranging from negative to positive values at various KCl concentrations. The rectifying degree ( R=I +V /I − V , where V =1.5 V) is plotted as a function of V G ( Fig. 5a ). The voltage tunability of the FERD devices (that is, the slope of the R-V G plot in Fig. 5a ) becomes less prominent at both high and low KCl concentrations. With 1 M and 100 mM KCl solutions, no diode characteristics (asymmetric I – V curve) were observed experimentally. The most pronounced voltage tunability happens at intermediate KCl concentrations (1 mM and 10 mM). The qualitative trend that the tunable rectifying property being most prominent at intermediate ion concentrations and weakened at both low and high ionic concentrations is also observed in the numerical calculations ( Supplementary Fig. S5 ). The rectifying degree shows a monotonically decreasing dependence on V G when [KCl]<100 mM. Consequently, the forward direction of the nanofluidic diode can be electrically switched by the application of an external gate potential (inset symbols of Fig. 5a ), consistent with the results in Figures 3 and 4 . 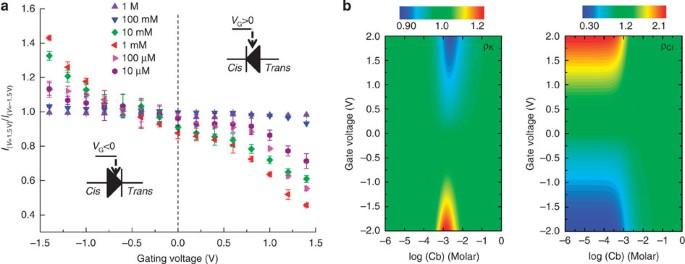Figure 5: Effect of the ionic concentrations on the rectifying degree under various gate potentials. (a) Experimental results. The error bars correspond to ten measurements. The inset symbols schematically show the forward direction switched with positive and negative gate voltages. (b) Calculated ratios of cation flux (ρK) and ratios of anion flux (ρCl) via theCisandTransside of the nanochannel as a function of gate potentialVGand bulk concentrationCb. The surface charge density used in the calculation is σs=−2 mC m−2. Figure 5: Effect of the ionic concentrations on the rectifying degree under various gate potentials. ( a ) Experimental results. The error bars correspond to ten measurements. The inset symbols schematically show the forward direction switched with positive and negative gate voltages. ( b ) Calculated ratios of cation flux ( ρ K ) and ratios of anion flux ( ρ Cl ) via the Cis and Trans side of the nanochannel as a function of gate potential V G and bulk concentration C b . The surface charge density used in the calculation is σ s =−2 mC m −2 . Full size image Another intriguing feature of Figure 5a is that, at a fixed gate voltage (for example, −1.5 V), the highest rectifying degree occurs at the intermediate ion concentrations rather than the lowest concentration regime where surface charge-governed ion conduction dominates. This counterintuitive phenomenon has also been observed in the systems of two terminal conical nanopore diodes [18] , and nanochannel diodes [20] , [21] , [22] , [24] , [41] . However, a physical picture is lacking in understanding this behaviour. Here we develop a physical model to explain these intriguing phenomena observed in our field-effect controlled diodes, with the aim to improve the rectification ratios. Referring to Figure 4a and considering the averaged concentrations of K and Cl ions at the two segments of the nanochannel, we denote the relation in the gated area (subscript C) and the un-gated area (subscript T) as [K] C = γ C [Cl] C , and [K] T = γ T [Cl] T , where γ is the cation/anion ratio. The cation/anion ratio can be determined through the electroneutrality and the law of conservation of mass as ( Supplementary Methods ), and , where S C =(2 σ s – ɛ 0 ɛ ox V g / d ox )/ ehN A and S T =2 σ s / ehN A . ɛ ox and d ox are the permittivity and the thickness of dielectric SiO 2 , respectively. By using the total current continuity at the micro/nano channel interfaces, we can obtain the ratios of cation (anion) flux via the Cis side over the cation (anion) flux via the Trans side of the nanochannel as ( Supplementary Methods ), To observe a rectifying behaviour, ρ K ≠1 and ρ Cl ≠1 are required in the nanochannels (that is, the two solid bars, or the two empty bars in Figure 4a should be unequal in length). In fact, the further the value of ρ K and ρ Cl deviates from unity, the more pronounced is the rectification. Apparently, ρ K or ρ Cl is a function of V G , C b and σ s , which is plotted in Figure 5b . At very high concentrations ( C b >100 mM), the averaged ion concentrations in the nanochannel are dominated by the bulk rather than the surface and, hence, are barely affected by the external potential. Therefore, γ C ≈1 and γ T ≈1 (bulk property), which results in ρ K = ρ Cl =1 and no rectifying behaviour would be observed. At very low concentrations ( C b <100ìμM), we obtain ρ K ≈1 and ρ Cl ≠1. However, since K is the majority carrier that dominates the total ionic flux, the rectifying effect is less significant. At intermediate concentrations ( C b ~1 mM), where ρ K ≠1 and ρ Cl ≠1, the most profound rectifying behaviour is expected. The above analysis implies the strategies that can be adopted to improve the gate-tunable rectifying effect. Higher rectifying effect will happen when γ C ≪ 1 ≪ γ T or γ T ≪ 1 ≪ γ C . For an intrinsically negatively charged nanochannel SiO 2 wall, it is obvious that γ T ≫ 1. To achieve γ C ≪ 1, the charge polarity beneath the gate electrode needs to be reversed, which requires ɛ 0 ɛ ox V g / d ox >2| σ s |. Take σ s =−2 mC m −2 , for example, the minimal gate voltage required for charge polarity reversal is about 9 V. This is inaccessible in our current devices owing to the gate leakage and breakdown limitations ( Supplementary Fig. S6 ). However, if a surround-gate architecture (that is, with both the top gate and the back gate) is used, the minimal gate voltage needed to reverse the charge polarity would be reduced by half. In addition, for a better control over cation/anion ratios, a low surface charge density is desirable. This is because an inherent high surface charge density in nanochannels resembles degenerate doping in a semiconductor or high surface state density of a FET, making the electrostatic control of the ionic concentrations in the nanochannel difficult [6] . By neutralizing the intrinsic surface charge through chemical modifications, it would allow for more efficient gate modulation in the Cis side. A separate gate on top of the Trans segment would further permit the cation/anion modulation in the Trans side. Therefore, by placing dual gate electrodes along the channel length, one can have more flexibility to tune the rectifying property via the dual gates. Moreover, reducing the nanochannel dimensions down to sub-10 nm would allow the diodes to function at a more realistic ionic concentrations (for example, physiological conditions, ~10–100 mM) [7] . To sum up, an ideal structure for field-effect reconfigurable nanofluidic diodes would be dual split-gates with a gate-all-around structure and a sub-10 nm nanochannels of a neutral surface. To experimentally verify these predictions, we fabricated another wafer of devices with a dual gate structure ( Fig. 6a ) and an 8-nm-thick nanochannel (determined by the thickness of the sacrificial Cr layer). The surface charge of the as-fabricated nanochannel is estimated as σ s =−1.6 mC m −2 ( Supplementary Fig. S7 ). This native surface charge density is reduced by sequentially treating the nanochannel wall with 3-Glycidoxypropyltrimethoxysilane and ethanolamine ( Supplementary Methods ). The resulting nanochannel surface is highly hydrophilic and the modified surface charge is estimated as σ s =−0.3 mC m −2 ( Supplementary Fig. S7 ). 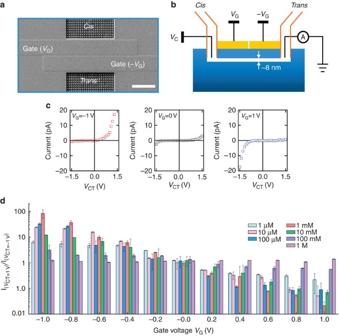Figure 6: Improved field-effect tunability over the ionic diode property with devices of a dual split-gate structure. (a) SEM image of the dual split-gate FERD devices (W=1 μm×11,L=116 μm,H=8 nm). The scale bar is 100 μm. The nanochannel wall is chemically modified to be less charged and hydrophilic. The separation between the two gates is 4 μm. (b) Testing configurations for the dual gate FERD device. (c) TypicalICT-VCTcurves at different gate voltagesVG(−1 V, 0 V, +1 V), for a given ionic concentration (1 mM). (d) Measured rectifying degree (referenced atVCT=±1 V) as a function ofVGfor KCl concentrations ranging from 1 μM to 1 M. With this surface-modified dual-gate device and an electrical setup schematically shown in Figure 6b , we recorded the I CT as a function of V CT for V G ranging from negative to positive values at various KCl concentrations. Figure 6c shows typical I CT -V CT curves at different gate voltages V G , for a given ionic concentration (1 mM). The rectifying ratio ( R=I +V /I −V , where V =1 V) is plotted as a function of V G for seven different KCl concentrations ( Fig. 6d ). The dual-gate device with the chemically modified surface shows a tremendously improved rectification ratio. At V G =−1 V, the rectification ratio reaches ~83 for 1 mM KCl, much higher than that of the single-gate device shown in Figure 5a (a ratio of ~1.2 under the same conditions). We note that the rectification ratio can be even higher under larger reference V CT biases. Interestingly, the dual-gate device also exhibits a higher rectifying degree at the intermediate ion concentrations under a fixed gate voltage (for example, V G =−1 V in Fig. 6d ). Figure 6: Improved field-effect tunability over the ionic diode property with devices of a dual split-gate structure. ( a ) SEM image of the dual split-gate FERD devices ( W =1 μm×11, L =116 μm, H =8 nm). The scale bar is 100 μm. The nanochannel wall is chemically modified to be less charged and hydrophilic. The separation between the two gates is 4 μm. ( b ) Testing configurations for the dual gate FERD device. ( c ) Typical I CT -V CT curves at different gate voltages V G (−1 V, 0 V, +1 V), for a given ionic concentration (1 mM). ( d ) Measured rectifying degree (referenced at V CT =±1 V) as a function of V G for KCl concentrations ranging from 1 μM to 1 M. Full size image In conclusion, we propose and demonstrate a field-effect reconfigurable nanofluidic diode based on an asymmetric field effect. This general concept could conceivably be applied to similar thin-body solid-state devices (for example, silicon-on-insulator or semiconducting nanowire). Compared with any existing nanofluidic control systems including stimuli-responsive tuning, the electrostatic modulation platform offers the full potential for logical programming of rectified transport of ionic and molecular species. Unlike the nanofluidic field-effect transistor, where only the amount of ions/molecules is regulated by an electrostatic potential, the FERD can be used to control both directions and magnitudes of ion/molecule transport. FERD represents a fundamentally novel system and may function as the building block to create an on-demand, reconfigurable, large-scale integrated nanofluidic circuits for digitally programmed manipulation of biomolecules such as polynucleotides and proteins. Device fabrication We used a sacrificial layer method to produce the nanochannels. However, there is a major difference in our process. The conventional method etches the sacrificial layer first and then integrates the nanochannel device with a microfluidic interface to form a functional device [22] , [24] , [42] . We find that the nanochannels fabricated by this method are inclined to collapse because of the capillary force in the drying process and/or the pressure exerted during the bonding process. To overcome this problem, we developed a novel 'bond-followed-by-etch' scheme. Briefly, 11 thin Cr stripes are patterned on top of an insulating SiO 2 layer on a 4-inch silicon wafer. Then a dielectric SiO 2 layer (50-nm-thick) is subsequently deposited by plasma enhanced chemical vapour deposition, followed by a rapid thermal annealing process to improve the dielectric quality. Gate electrode is thereafter formed by a double layer lift-off process. The accessing reservoirs with supporting pillars are etched simultaneously by reactive CHF 3 /Ar plasma at a rate of 1 nm s −1 . The device is then aligned and permanently bonded with a microfluidic polydimethylsiloxane stamp. The Cr etchant is pumped into the microchannel afterwards, which diffusively etches the Cr sacrificial layer in situ . The end-point detection for the etching process is done by looking at the colour contrast under a microscope. Deionized water is flushed through the microchannel after the etching process is finished, and then the device is ready to use. As neither the drying process nor the external pressure is applied, the 'bond-followed-by-etch' scheme completely avoids the nanochannel collapse problem. Moreover, the top-down process results in a uniform nanochannel dimensions along the length the channels and across the array. Electrical characterization The whole testing procedure is done using an automatic system. The solutions are delivered by pumps (New Era Pump Systems), controlled by a LabVIEW program (National Instruments). The current-voltage measurement is performed using HP4156B semiconductor parameter analyzer and is synchronized with the pump by the same LabVIEW program. Data post-processing is done with MATLAB (The MathWorks) software. Numerical calculation The steady-state distributions of the cation/anion concentration and the ionic current under different V G and V CT biases are calculated by solving the coupled two-dimensional Poisson–Nernst–Planck equations within the COMSOL script environment. We use three modules in the COMSOL environment: Electrostatics (AC/DC Module), Nernst–Planck without electroneutrality for the calculation of K + ions (Chemical Engineering Module) and Nernst–Planck without electroneutrality for the calculation of Cl − ions (Chemical Engineering Module). The simulation system contains an 8-μm-long, 20-nm-high nanochannel that is connected by two 1×1 μm 2 square reservoirs. The SiO 2 dielectric is 50-nm-thick and 4-μm-long, with surface charge density as σ s =−2 mC m −2 . The length of the nanochannel used for calculation is less than the real device (100 μm) to reduce the simulation time. How to cite this article: Guan W. et al . Field-effect reconfigurable nanofluidic ionic diodes. Nat. Commun. 2:506 doi: 10.1038/ncomms1514 (2011).